Structural and functional differences in medial prefrontal cortex underlie distractibility and suppression deficits in ageing Older adults experience deficits in working memory (WM) that are acutely exacerbated by the presence of distracting information. Human neurophysiological studies have revealed that these changes are accompanied by a diminished ability to suppress visual cortical activity associated with task-irrelevant information. Although this is often attributed to deficits in top-down control from a prefrontal cortical source, this has not yet been directly demonstrated. Here we evaluate the neural basis of distraction’s negative impact on WM and the impairment in neural suppression in older adults by performing structural and functional MRIs while older participants engage in tasks that require remembering relevant visual stimuli in the context of overlapping irrelevant stimuli. Analysis supports both an age-related distraction effect and neural suppression deficit, and extends our understanding by revealing an alteration in functional connectivity between visual cortices and a region in the default network, the medial prefrontal cortex (mPFC). Moreover, within the older population, the magnitude of WM distractibility and neural suppression are both associated with individual differences in cortical volume and activity of the mPFC, as well as its associated white-matter tracts. Interactions with the external environment involve engaging with multiple, competing sensory stimuli [1] , [2] . Goal-directed, attentional mechanisms orient our limited cognitive resources towards task-relevant information and away from task-irrelevant, distracting stimuli [3] . Previous studies have shown that as we age, individuals become increasingly susceptible to a negative impact of distracting information on a diverse set of performance measures, suggesting a diminished capacity to effectively filter task-irrelevant stimuli (that is, the inhibitory deficit hypothesis) [4] . Working memory (WM) is the ability to hold and manipulate information in mind to guide subsequent behaviour [5] . Consistent with the inhibitory deficit hypothesis, older adults often experience greater impairment in WM performance in the presence of irrelevant, distracting information [6] , [7] , [8] . When an individual is presented with task-irrelevant stimuli, the neural representation of this information in stimulus-selective visual cortices is suppressed via top-down control mechanisms [9] , [10] . The prefrontal cortex has been established as a source of this goal-directed, top-down modulation of activity in sensory cortex that serves to bias subsequent WM performance [11] . Older adults exhibit a selective deficit in the suppression of sensory-based neural activity to irrelevant information that is predictive of their WM performance declines [6] . Despite the many studies characterizing this age-related top-down suppression deficit [12] , [13] , [14] , the underlying neural mechanisms—notably the role of the prefrontal cortex—and the basis for individual differences within the older population that mediate the impact of distraction on WM performance remain elusive. The primary goal of this study was to explore how individual differences in the structure and function of prefrontal cortical control regions—particularly those linked to the process of neural suppression—relate to differences in suppression and WM distractibility within a population of older adults. Recent evidence in younger adults revealed that a network of distributed cortical regions that are deactivated during cognitively demanding tasks (that is, the default network [15] , [16] , notably the medial prefrontal cortex (mPFC)) are functionally coupled to visual areas that selectively process irrelevant visual stimuli [9] . Moreover, functional connectivity between mPFC and visual cortex is predictive of the degree of neural suppression and WM distractibility in younger adults. Since the mPFC seems to play a vital role in the active suppression of task-irrelevant information, we hypothesized that a functional disconnection between mPFC and visual cortical regions modulates the age-related selective suppression deficit. Although age-related alterations in the function of the default network, such as the mPFC, have been reported [17] , [18] , a link has not yet been established with neural suppression abilities or WM distractibility in older adults. In the current study, healthy older adults (60–85 years) engaged in a selective-attention, WM paradigm during a magnetic resonance imaging (MRI)-recording session. Both univariate and functional connectivity fMRI data were directly compared with a previously collected data set from younger adults (18–35 years) [9] . Moreover, high-resolution structural and diffusion-tensor imaging (DTI) data were acquired to probe neural and behavioural relationships within the older group, specifically assessing whether individual differences in grey-matter volume and white-matter integrity correlate with measures of neural suppression and WM distractibility in older adults. The experimental paradigm involved five conditions presented in blocks ( Fig. 1 ). In two WM conditions, sequential images of two faces or two scenes were presented (that is, no distraction) and participants were instructed to remember both stimuli over a short delay period and then respond to a memory probe (face memory (FM) or scene memory (SM)). In the remaining three conditions, the stimuli consisted of transparent faces overlapped with transparent scenes. Instructions before each block designated which stimuli should be remembered, with the other stimuli serving as distractors (FM-overlap (FM-O), SM-overlap (SM-O)) or if the overlapping stimuli should be passively viewed with no memory goals (passive-view-overlap (PV-O)). The advantage of this design is that neural indices of top-down suppression of visual cortical activity to irrelevant stimuli (‘suppression’) can be extracted by contrasting activity measures from the overlap WM conditions with the overlap passive-view condition, and behavioural indices of the impact of distraction on WM performance (‘distractibility’) can be obtained by comparing accuracy on overlap WM conditions with non-overlap WM conditions [9] , [19] . Results converge to show that distractibility and suppression deficits in older adults stem from individual differences in the structure and function of the mPFC. 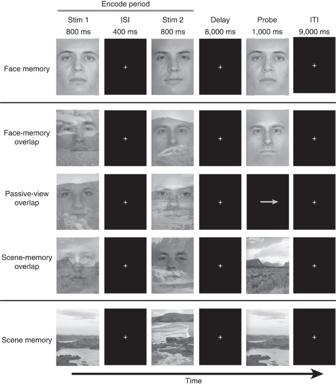Figure 1: Experimental paradigm. Participants were instructed to remember both Stim1 and Stim2, then respond with a button press if the probe image matched either of the previous relevant stimuli. Participants were instructed to maintain fixation on the white crosshairs9. Figure 1: Experimental paradigm. Participants were instructed to remember both Stim1 and Stim2, then respond with a button press if the probe image matched either of the previous relevant stimuli. Participants were instructed to maintain fixation on the white crosshairs [9] . Full size image Age-related changes in distractibility To investigate age-related changes in WM performance, accuracy and response time (RT), data were subjected to a 2 × 2 × 2 analysis of variance (ANOVA) with age (younger and older), distraction (overlap and non-overlap) and stimulus (faces and scenes) as factors. 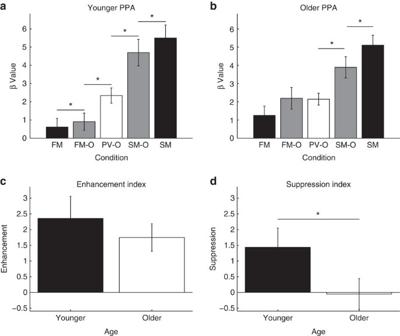Figure 2: Stimulus-selective visual association cortex activity. The encode-period activity in the left parahippocampal place area (PPA) for, (a) younger and (b) older adults. (c) Comparison of younger (black bars,n=22) and older (white bars,n=18) adult enhancement indices (SM-O–PV-O). (d) Comparison of younger and older adult suppression indices (PV-O–FM-O), revealing a selective suppression deficit in older adults. Error bars are s.e., *P<0.05. Analysis of accuracy data revealed a main effect of age (F(1,38)=12.36, P <0.001), such that younger participants showed significantly better WM performance (that is, increased accuracy) compared with older participants ( Supplementary Table 2 ; Supplementary Fig. 1A ). In addition, there was a main effect of distraction (F(1,38)=108.11, P <0.0001), such that participants exhibited better WM performance on conditions when stimuli were not overlapped (FM and SM) compared with conditions with overlapped stimuli (FM-O and SM-O). No main effect of stimulus type (that is, faces versus scenes) was observed (F(1,38)=1.72, P =0.2). Furthermore, there was no significant interaction between distraction and age (F(1,38)=1.46, P =0.2) and there were no other significant interactions for accuracy data (each P >0.2). For the ANOVA of correct-only RT, main effects were significant for both age (F(1,38)=4.08, P <0.05) and distraction (F(1,38)=72.37, P <0.0001), such that older participants responded more slowly for all conditions compared with younger adults and the participants’ responses were slowed by the presence of overlapped, distracting stimuli. No significant effect was observed for stimulus type (F(1,38)=3.33, P =0.1). In contrast to accuracy data, a significant interaction was observed between age and distraction (F(1,38)=4.07, P <0.05), such that older adults showed a significantly greater impact of distraction on RT in the overlapped conditions versus non-overlapped conditions compared with the older adults ([FM-O+SM-O]–[FM+SM]; t(38)=2.02, P <0.05). That is, older adults disproportionately slowed their responses in the setting of distraction relative to young adults, revealing the presence of an age-related distraction effect that impacted WM performance by delaying the speed of recognition. No other significant interactions for RT were observed (each P >0.2). Age-related changes in suppression To evaluate age-related changes in the top-down modulation of visual processing, activity measures were derived by modelling-encoding period activity using a general linear model (GLM). Parameter estimates (beta values) were computed for correct trials only from a scene-selective region of interest (ROI), the left parahippocampal place area (PPA) [20] , which has been shown to be the most robustly activated visual cortical region for scene stimuli [6] , [9] , [10] . Note that the face-fusiform area (FFA) was not evaluated in this study, as even younger adults do not consistently display suppression in this region (shown in previous reports [6] , [9] , [10] ) and thus the FFA does not serve as a useful region to explore age-related changes in suppression. In the PPA of younger participants, the data revealed that scene stimuli presented in isolation induced significantly greater activity than face stimuli presented in isolation (bottom-up, stimulus-driven effect) (SM>FM: t(21)=7.12, P <0.0001) ( Fig. 2a ). In addition, there was a significant effect of top-down modulation, such that all three overlapped conditions revealed significantly different levels of activation depending on task goals: enhancement of PPA activity when scenes were relevant compared with passive-view baseline (SM-O>PV-O; t(21)=3.33, P <0.005), and significant suppression of PPA activity when scenes were irrelevant compared with baseline (FM-O<PV-O; t(21)=2.34, P <0.05). These three levels of activation (SM-O>PV-O>FM-O) represent a pure, top-down effect because bottom-up information was constant throughout the task. Moreover, the magnitude of the effects for the overlapped conditions fell between the levels attained in pure conditions (SM>SM-O>PV-O>FM-O>FM, P <0.05). Figure 2: Stimulus-selective visual association cortex activity. The encode-period activity in the left parahippocampal place area (PPA) for, ( a ) younger and ( b ) older adults. ( c ) Comparison of younger (black bars, n =22) and older (white bars, n =18) adult enhancement indices (SM-O–PV-O). ( d ) Comparison of younger and older adult suppression indices (PV-O–FM-O), revealing a selective suppression deficit in older adults. Error bars are s.e., * P <0.05. Full size image PPA data from the older participants also showed selectivity for scenes (SM) compared with faces (FM), such that scenes elicited a greater response ( Fig. 2b ; SM>FM: t(17)=7.95, P <0.0001), displaying the bottom-up selectivity of this region. In addition, older participants demonstrated neural enhancement when overlapped scenes were task-relevant compared with passive (SM-O>PV-O: t(17)=3.96, P <0.001). However, there was no significant top-down suppression when scenes were task-irrelevant compared with passive (FM-O<PV-O: t(17)=0.10, P =0.9). Since the current experimental paradigm included a direct measure of PPA bottom-up stimulus selectivity (that is, SM versus FM), the top-down effects (SM-O versus PV-O versus FM-O) can be normalized by each participant’s stimulus selectivity. When the measure of suppression (PV-O–FM-O) was expressed as a percentage of stimulus selectivity (SM–FM) there was still no significant level of suppression for older participants (t(17)=0.76, P =0.5), while enhancement was significant (t(17)=2.27, P <0.05). Univariate data from the PPA were directly compared between younger and older participants using a 2 × 3 ANOVA with age and conditions (overlapped stimuli FM-O, PV-O and SM-O) as factors. Analysis revealed a main effect of condition (F(2,76)=27.23, P <0.0001), but not of age (F(2,38)=0.02, P =0.9). However, a significant interaction was observed between age and condition (F(2,38)=3.59, P <0.03). Post hoc analysis revealed that younger and older participants did not show significant differences in enhancement at the group level ( Fig. 2c , SM-O>PV-O: t(38)=−0.68, P =0.5), even when normalized for differences in bottom-up selectivity (t(38)=−0.45, P =0.7), but did show different degrees of suppression, such that younger participants showed significantly greater suppression than older participants ( Fig. 2d , t(38)=1.83, P <0.05). This finding is consistent with previous studies demonstrating a selective age-related suppression deficit, wherein older participants exhibited diminished suppression of task-irrelevant visual stimuli in the setting of preserved enhancement [6] . Importantly, this age-related selective suppression deficit exists even when normalized for differences in bottom-up stimulus selectivity (t(38)=1.92, P <0.05), demonstrating that the observed effect is not driven by a loss of visual association cortex selectivity in ageing [21] . Age-related changes in the suppression network To investigate age-related changes in functional brain networks that are associated with neural suppression (‘the suppression network’), functional connectivity maps were generated and compared across age groups. Capitalizing on trial-by-trial variability, whole-brain functional connectivity maps were assessed by correlating activity from the left PPA seed region with voxels from the rest of the brain [22] , [23] . Regions that are highly correlated with a seed region across trials are presumed to be functionally connected, thereby defining large-scale networks associated with activity modulation within those regions. A suppression network map was generated by contrasting the PPA connectivity maps obtained from the FM-O and PV-O conditions (that is, comparing the condition when scenes were task-irrelevant to the condition when there were no top-down attentional demands) [9] , [24] . As previously reported in younger participants, the suppression network (FM-O>PV-O) includes the mPFC, posterior cingulate cortex (PCC), retrosplenial cortex and bilateral parietal cortex (PC), which overlaps with the classically described default network [9] ( Fig. 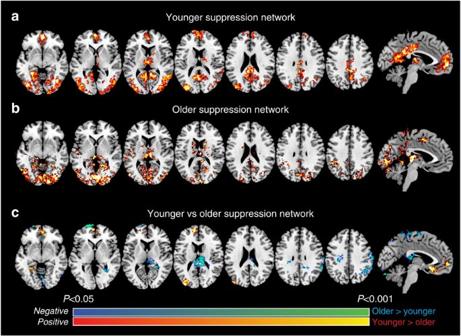Figure 3: Younger versus older suppression network. (a) Functional connectivity map for younger participants (n=22) using a PPA seed, contrasting FM-O>PV-O (that is, suppression network). (b) Same asa, but for older participants (n=18). (c) Contrast between younger and older suppression network maps. All images thresholded atP<0.05 and are corrected for multiple comparisons using the cluster method described in Methods. 3a ; Supplementary Table 3 ). However, this same analysis in older participants did not reveal the mPFC to be a node in the suppression network, although PCC and, to some extent, bilateral PC connectivity were present ( Fig. 3b ; Supplementary Table 3 ). A difference in PPA-mPFC connectivity between younger and older participants was confirmed to be significant by a whole-brain contrast between younger and older data ( Fig. 3c ; Supplementary Table 3 ). PCC and right PC functional connectivity with the PPA did not show age-related differences, although the left PC did. Interestingly, older adults did show a significant increase in functional connectivity between the PPA and supplementary motor area and the PPA and left superior parietal lobule. These network changes may represent a compensatory mechanism in the older brain, which is insufficient to prevent a decline in suppression abilities. Figure 3: Younger versus older suppression network. ( a ) Functional connectivity map for younger participants ( n =22) using a PPA seed, contrasting FM-O>PV-O (that is, suppression network). ( b ) Same as a , but for older participants ( n =18). ( c ) Contrast between younger and older suppression network maps. All images thresholded at P <0.05 and are corrected for multiple comparisons using the cluster method described in Methods. Full size image These results demonstrate that in addition to the suppression deficit in older participants, the suppression network is significantly altered in ageing, notably the coupling between the mPFC and visual cortices representing irrelevant stimuli. Age-related changes in the default network The default network is a collection of regions that are deactivated during attentionally demanding tasks and have been associated with ‘internalized thought’ processes, such as mind-wandering and introspection [15] , [16] , [25] , [26] . Interestingly, the default network has been shown to exhibit functional changes in ageing [17] , [27] , [28] . Relevant to the goals of this study, it has been demonstrated that brain regions of the default network (notably the mPFC and PCC) are functionally connected with visual cortical regions in a manner predictive of the degree of suppression of irrelevant information in the stimulus-selective visual cortex (that is, in the PPA) [9] . Here, we evaluated age-related changes within the default network to assess whether these changes are consistent with our observed reduction in mPFC/visual cortical functional connectivity. Default network activity modulation was derived using an independent task, distinct from the main experimental paradigm (see Methods), in both the younger and older adults, that assessed deactivation patterns during an attentionally demanding visual n-back task relative to rest [15] , [16] , [25] ( Fig. 4 ). 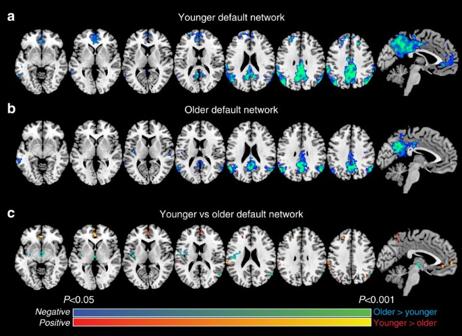Figure 4: Younger versus older default network. (a) Whole-brain analysis showing regions with significantly greater activity at rest during independent task (rest>task) for younger participants (n=22). (b) Same asa, but for older participants (n=18). (c) Contrast between younger and older participants’ default network maps. All images thresholded atP<0.05 and are corrected for multiple comparisons using the cluster method described in Methods. Figure 4: Younger versus older default network. ( a ) Whole-brain analysis showing regions with significantly greater activity at rest during independent task (rest>task) for younger participants ( n =22). ( b ) Same as a , but for older participants ( n =18). ( c ) Contrast between younger and older participants’ default network maps. All images thresholded at P <0.05 and are corrected for multiple comparisons using the cluster method described in Methods. Full size image Whole-brain analysis of the younger participants revealed the canonical set of default network regions [15] , [16] , [25] , with deactivation of mPFC, PCC and bilateral PC ( Fig. 4a ), while older participants exhibited deactivation within several nodes of the default network (that is, PCC and bilateral PC), but no significant deactivation of the mPFC ( Fig. 4b ). An across-age-group contrast supported the conclusion that older adults deactivate areas of the default network less than younger adults, consistent with previous studies [18] , [28] ( Fig. 4c ). Note that this independent analysis further positions the mPFC as an area of interest for age-related attentional changes, which parallels the age-related change in functional connectivity between the mPFC and the PPA during the selective-attention, WM task ( Fig. 3c ). It should be noted that this analysis of default network activity identified age-based declines in an mPFC region (center of mass in Montreal Neurological Institute (MNI) coordinates [−2 50 4]) that has 25.4% overlap with the age-based decline in mPFC activity identified by the suppression network analysis (center of mass in MNI coordinates [−4 58 0]). Therefore, these separate analyses converge to show age-related declines in a common subregion of the mPFC (overlapping center of mass MNI coordinates [−4 56 4]). To address whether the precise location of these age-related changes in mPFC are consistent with previous reports of mPFC involvement in the default network, an mPFC ROI was created (7 mm radius sphere centered at Talairach coordinates [1 40 16]) from a previous report of age-related declines in default-mode activity [29] . Default mode activity was averaged within this mPFC ROI for each participant and compared between the two age groups. Confirming our previous analyses, older adults exhibited less mPFC default mode deactivation (t(38)=2.22, P <0.05). This result extends our previous findings and show consistency with prior reports regarding the mPFC location of an age-related decline in default mode processes. Relationship between distractibility and suppression To capitalize on within-group heterogeneity of the older population to explore relationships between individual differences in performance and neural measures, across-participant regression analyses were performed between the magnitude of suppression (PPA activity in PV-O–FM-O) and distractibility (WM accuracy in FM–FM-O) in the older cohort. This analysis revealed a significant negative correlation ( Fig. 5 : r =−0.70, P <0.001), such that those individuals who least suppressed the irrelevant scenes exhibited the greatest impact of distraction on WM accuracy for faces. No similar relationship was revealed for WM RT ( r =−0.01, P <0.99). This result supports previous data showing that successful suppression is critical for distraction-resistant memory in older adults [6] , [12] , [14] , [30] . This correlation was not significant in younger participants ( r =−0.22, P =0.3), consistent with previous studies [6] , [10] , and was significantly different across age groups ( P <0.05). However, this may be due to near-ceiling performance in younger adults, as a relationship between WM performance and top-down modulation of visual cortical activity has been shown in other studies of younger adults [19] , including a relationship specific to suppression [31] . 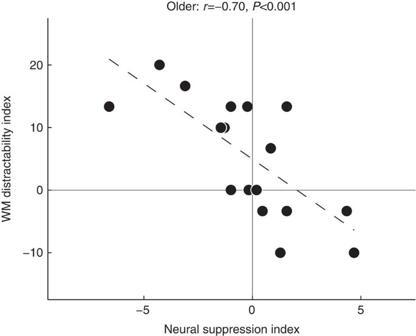Figure 5: Neural behavioural correlation. Relationship between WM distractibility (accuracy in FM–FM-O) and neural suppression in older adults (n=18). *P<0.001. Figure 5: Neural behavioural correlation. Relationship between WM distractibility (accuracy in FM–FM-O) and neural suppression in older adults ( n =18). * P <0.001. Full size image To assess whether the age-related decline in PPA suppression is reflective of a more general cognitive decline, additional across-participant regression analyses in older adults were conducted between the magnitude of suppression and neuropsychologial data (listed in Supplementary Table S1 ). This analysis revealed no significant correlations between PPA suppression and data from any neuropsychological test (each comparison P >0.5, corrected). This suggests that age-based declines in task-related WM performance are more likely attributed to a selective suppression deficit to distraction rather than generalized cognitive changes. Gray matter relationship with distractibility and suppression Older adults exhibit reduced grey-matter volume and thickness compared with healthy, younger adults [32] , [33] , [34] , which have been shown to relate to cognitive impairment [35] , [36] . We used voxel-based morphometry (VBM) [37] , [38] and whole-brain, across-participant regression analyses to assess the relationship of grey-matter volume with distractibility and suppression in older individuals. The WM distractibility data demonstrated a prominent correlation with the volume of grey matter in the mPFC (corrected for multiple comparisons), such that older adults with the least mPFC grey-matter volume (MNI coordinates: [−2, 62, 14]) exhibited the greatest impact of distraction on WM performance ( Fig. 6a ). The suppression analysis also revealed a parallel finding, such that reduced cortical volume within the mPFC (MNI coordinates: [2, 62, 2]) was associated with reduced suppression of activity within the PPA in the presence of irrelevant scenes ( Fig. 6b ). Although we report different coordinates for the center of mass of these mPFC clusters, there is significant overlap between these mPFC regions at the group level. Taken together, these results reveal a dependency on cortical volume of the mPFC in older adults to resist the negative influence of distraction on WM performance, as well as to effectively engage top-down suppression mechanisms. Interestingly, although the mPFC is one of several nodes comprising the canonical default network, it was the only default network region that was revealed in these analyses. 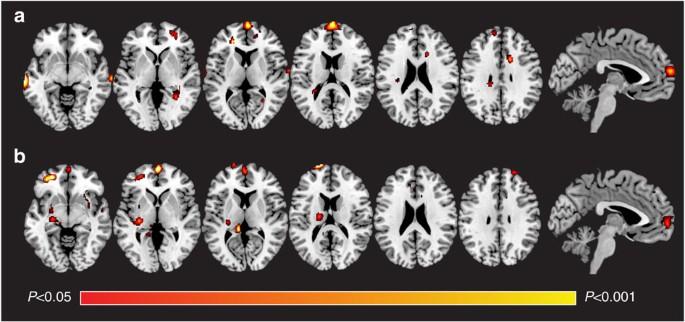Figure 6: Gray-matter volume. Relationship with (a) WM distractibility and, (b) neural suppression in older participants (n=18). All images thresholded atP<0.05, corrected for multiple comparisons. Figure 6: Gray-matter volume. Relationship with ( a ) WM distractibility and, ( b ) neural suppression in older participants ( n =18). All images thresholded at P <0.05, corrected for multiple comparisons. Full size image White matter relationship with distractibility and suppression Changes in the integrity of white-matter pathways have been observed to occur in normal ageing [39] , [40] and are associated with age-related cognitive deficits [29] . To investigate the relationship between white matter and distractibility and suppression across older individuals, DTI data were acquired and processed using a tract-based spatial statistical (TBSS) approach to analyse the fractional anisotropic (FA) data [41] , [42] . When TBSS-normalized FA data were regressed against the WM distractibility index, a significant correlation was found with several white-matter tracts, such that older adults with the lower FA (that is, decreased white-matter integrity) in prefrontal calossal fibres were more susceptible to the negative impact of distracting stimuli on WM performance ( Fig. 7a ). This frontal white-matter tract has previously been shown to be associated with age-related cognitive decline [43] , [44] , [45] , [46] . White-matter integrity was also positively correlated with suppression indices in the superior longitudinal fasciculus in the older adults, such that those participants with lower FA levels exhibited lower levels of suppression ( Fig. 7b ). Interestingly, this pathway lies between the mPFC and PCC (two regions of the suppression and default networks). Moreover, decreased superior longitudinal fasciculus integrity has been shown to be correlated with decreased executive function and default network function in older adults [29] . 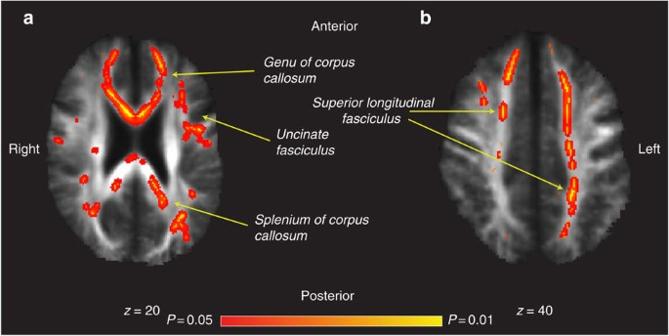Figure 7: White-matter integrity. Relationship with (a) WM distractibility and, (b) neural suppression in older participants (n=18). All images are corrected for multiple comparisons and displayed atP<0.05. Figure 7: White-matter integrity. Relationship with ( a ) WM distractibility and, ( b ) neural suppression in older participants ( n =18). All images are corrected for multiple comparisons and displayed at P <0.05. Full size image Suppression network relationship with distractibility and suppression An analysis to investigate whether the degree of functional connectivity within the suppression network was predictive of distraction and suppression levels revealed no significant correlation in older adults. Interestingly, previous results demonstrated that functional coupling between the mPFC and the PPA in the setting of suppression was predictive of the magnitude of both WM distractibility and suppression in younger adults [9] . This relationship was seemingly disrupted in older participants, that is, increased PPA-mPFC coupling was not predictive of an older participant’s degree of PPA suppression (no regions survived a whole-brain analysis using P <0.05 threshold, corrected for multiple comparisons). Default network relationship with distractibility and suppression To evaluate whether age-related dysfunction of activity modulation in the default network was related to the described neural and performance distraction effects on the WM task, across-participant regression analyses was performed between WM task-induced mPFC suppression (measured via the index: PV-O activity–FM-O activity) and distractibility and suppression indices for each age group. The distractibility analysis revealed a significant relationship in older adults, such that those individuals who exhibited less task-induced mPFC suppression showed a greater impact of distraction on WM performance ( Fig. 8a : r =−0.50, P <0.03). This relationship was not significant in younger participants ( r =−0.23, P =0.3) but did not significantly differ between age groups ( P =0.1). For the suppression analysis, older adults again showed a significant relationship, such that those participants who exhibited less mPFC suppression also showed less PPA suppression ( Fig. 8b : r =0.54, P <0.02). This correlation was also not significant in younger adults ( r =0.14, P =0.5), but was not significantly different between age groups ( P =0.1). Taken together, these results demonstrate a link between mPFC function, WM distractibility distraction and PPA suppression in older adults. 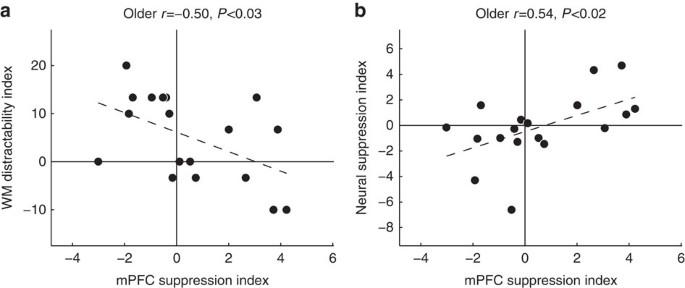Figure 8: Neural correlates. Relationship between mPFC activity suppression and (a) WM distractibility and (b) neural suppression within the PPA for older participants (n=18).P<0.03 andP<0.02, respectively. Figure 8: Neural correlates. Relationship between mPFC activity suppression and ( a ) WM distractibility and ( b ) neural suppression within the PPA for older participants ( n =18). P <0.03 and P <0.02, respectively. Full size image The present study was designed to identify an underlying structural and functional neural basis for the impact of distraction on WM performance and the deficit in top-down suppression of irrelevant information experienced by older adults. Our analytical approach involved a series of across-age-group comparisons and within-group regression analyses of MRI and behavioural measures to capitalize on individual differences between older adults. Several age-related changes consistent with previous studies were revealed: older adults exhibited: (1) WM impairment [47] , (2) a more negative influence of irrelevant information on WM performance [12] , (3) a deficit in the suppression of activity in visual cortical regions representing irrelevant information [6] and (4) a diminished ability to suppress activity in the mPFC default network region in response to an attentionally demanding task [1] , [17] , [18] , [27] , [28] , [48] . In addition, consistent with previous findings, older adults who exhibited less suppression of visual cortical activity associated with task-irrelevant information experienced a more negative impact of distraction on WM performance [6] , [12] , [14] . Importantly, several novel results were obtained: (1) older adults exhibited an alteration in functional connectivity of the suppression network relative to younger adults, notably a lack of coupling between visual association cortex and mPFC. (2) Those older adults with diminished task-induced mPFC suppression exhibited less suppression of irrelevant face information in the PPA and a greater impact of distraction on face WM performance. (3) The magnitude of both PPA activity suppression and WM distractibility were correlated with grey-matter volume of the mPFC, such that older adults with lower volume showed greater WM distractibility and lower levels of suppression. (4) A similar relationship was observed for white-matter integrity in prefrontal regions, such that reduced FA values in these pathways were correlated with increased WM distractibility and decreased suppression. Together, these results reveal a novel association between structural, functional and behavioural measures in older adults, providing converging evidence that anatomical and physiological differences between older individuals in the mPFC, and associated fibre tracts, are associated with the impact of distraction on WM and the neural suppression of irrelevant information. One prominent view of cognitive ageing maintains that older adults exhibit a diminished ability to filter task-irrelevant, distracting information (inhibitory deficit hypothesis) [4] , [49] , [50] . Results from previous experiments from our lab using sequentially presented face and scene stimuli, offered a neurophysiological basis for this hypothesis by revealing a selective suppression deficit in stimulus-selective visual cortices of older adults [6] . Using electroencephalography, we have shown that the suppression deficit occurs at very early stages of visual processing [14] , even if predictive information [13] or extra time to prepare for a distractor [12] was available. Here, we extend these findings by showing that the suppression deficit is present in older adults even when they are confronted with distracting stimuli that spatially and temporally overlap with task-relevant stimuli. This shows that simultaneous demands for visual-processing resources that likely engage biased-competition mechanisms of suppression [51] , [52] do not resolve this age-related deficit. The design of the present study further clarified the top-down nature of the suppression deficit. Others have revealed that visual cortical areas become less stimulus-selective in older adults [21] . Although it seems unlikely that such a change would be the basis of a selective deficit in suppression that occurs in the setting of preserved neural enhancement of relevant information, this possibility could not be directly assessed with previous data sets [6] . In the current study, conditions were included that contained no distracting information (FM and SM). Thus, top-down effects (FM-O versus PV-O versus SM-O) could be normalized for bottom-up differences in stimulus representation (FM versus SM) to determine whether the age-related suppression deficit occurred through top-down mechanisms. Analysis revealed that the suppression deficit was observed even when normalizing for stimulus-processing levels in the absence of distraction, supporting the conclusion that the age-related suppression deficit is due to changes in top-down modulation. Of note, WM RT exhibited differences in distractibility between age groups while WM accuracy correlated with PPA suppression in older adults. Although this could reflect how different types of variance influence statistical test results (that is, across-group ANOVA versus within-group regression), it might be argued that accuracy and RT reflect independent aspects of WM performance, thereby creating a distinction between the observed PPA suppression deficit in older adults and age-related declines in WM performance. To address this, a regression analysis was conducted across all participants between distractibility measures of accuracy and RT. Results showed a significant correlation between these measures ( r =0.31, P =0.05), supporting previous reports that suggest accuracy and RT are not independent measures of WM performance [53] , [54] . Moreover, it should be noted that both age groups exhibited declines in WM accuracy due to distraction, and that older adults were less accurate overall. Therefore, older adults may have disproportionately slowed their responses in the setting of distraction in order to maintain accuracy, which was already deficient relative to younger adults. Importantly, the present results offer novel evidence for a role of the mPFC in distractibility and suppression abilities in older adults: (1) An age-related alteration in the suppression network prominently involves the mPFC ( Fig. 3 ; Supplementary Table 3 ); (2) activity regulation in regions of the default network, notably the mPFC, is compromised in ageing ( Fig. 4 ); (3) activity suppression in this region predicts WM distractibility and neural suppression of irrelevant information in older adults ( Fig. 8 ); and (4) The structural integrity of the mPFC and its white-matter connections are associated with individual differences in inhibitory abilities in the older population: that is, across-participant regression analysis revealed significant correlations between WM distractibility and neural suppression, and mPFC grey-matter volume ( Fig. 6 ) and FA in underlying white matter ( Fig. 7 ). Although these data are correlational and do not address whether structural changes in ageing are causal of observed functional and behavioural effects, we hypothesize that grey- and white-matter structural changes precede functional changes and that this induces performance alterations; that is, increased distractibility. Of note, we are not claiming that the role of the mPFC in these processes is the result of the ageing process. Indeed, we have previously demonstrated a role of the mPFC in distractibility and suppression of irrelevant information in younger adults [9] . In the context of other studies that have shown the mPFC and underlying white matter are sensitive to age-related changes [18] , [29] , [33] , [55] , [56] , we hypothesize that alterations in the integrity of this region and its distributed networks occurs to varying degrees in older individuals resulting in a suppression deficit and greater distractibility compared to younger adults. Future research will be conducted to understand the root cause of the individual variability. In addition, exploring the progression from structural to functional to behavioural changes is critical for a comprehensive characterization of age-related cognitive changes and may be best accomplished via longitudinal studies. Although these data reveal a novel role of the mPFC in cognitive ageing, alterations in this brain region in older adults have been reported. From a functional perspective, there are consistent descriptions that older individuals do not suppress mPFC activity during externally directed tasks to the same degree as younger adults, most notably during more demanding tasks, and this has been associated with performance deficits on those tasks [18] , [27] , [28] , [48] , [57] . These mPFC changes are often considered to be reflective of more widespread, age-related default network dysfunction [58] . Functional connectivity between the mPFC and other regions of the default network during tasks are reduced in older adults [17] , and this has been related to disrupted cognitive performance [57] and compromised white-matter integrity [29] . Consistent with this, the default network as assessed by resting state functional connectivity is also diminished in ageing [61] , and this is associated with cognitive deficits [59] , although this may depend on the method used [60] . The current findings are supportive of these emerging trends in the literature that reveal functional and structural dysfunction of the mPFC and its network connections in older adults, and extend them to deficits in the critical domain of inhibitory function (both neural measures and behavioural consequences). A role of the mPFC in the age-related suppression deficit is consistent with recent findings that this region serves as a prominent node of the suppression network in younger adults, and that the degree of functional coupling between the mPFC and visual cortices is predictive of the neural suppression of task-irrelevant information. Accumulating evidence suggest that the default network is related to introspective or internalized cognitive processes, such as mind wandering [26] , [61] and retrospective and prospective memory [15] , [26] , [62] . Activity in default network, notably the mPFC [63] , is increased during these processes [26] , [61] , while they are deactivated during externally directed tasks [9] , [17] , [18] , [25] , [27] , [28] , [64] , possibly to reduce the negative impact of internal distraction. Consistent with this notion, studies have found that the degree of deactivation and fidelity of this network in ageing is predictive of performance [17] , [29] , [65] . We interpret the finding of a relationship between the suppression network and default network in younger adults, characterized as correlated activity modulation between mPFC and visual cortical areas that represent irrelevant stimuli, as evidence that suppression of external, distracting stimuli is coupled to the inhibition of internally generated, distracting thoughts [9] . In other words, a common mode of suppression is engaged for interference with task goals, whether it is present in the internal or external environment. The current finding suggests that dysfunction of the default network in ageing, particularly the mPFC, is associated with a disturbance of this relationship, resulting in greater WM distractibility and impaired neural suppression in agreement with others [66] . The results of the present study support previous reports that demonstrate successful suppression of task-irrelevant information is associated with better WM performance in both younger and older adults [6] , [31] . Here we provide evidence linking individual differences in mPFC function and structural integrity with this relationship in older adults. More generally, these results serve to bridge the literature of inhibitory deficits and default network dysfunction in older adults. Participants Functional and high-resolution anatomical MRI images were obtained from 23 healthy younger participants (ages: 18–34 years, mean: 23.7, females: 11) and 20 healthy, older participants (ages: 62–81 years, mean: 70.8, females: 11) while performing the task described below (see Supplementary Table 1 ). Participants were recruited, gave informed consent and compensated monetarily as per the UCSF Committee on Human Research approval. All participants had normal or corrected-to-normal vision and were taking no psychotropic medications. Experimental conditions were held constant for both participant groups (that is, same scanning parameters, stimuli-sets and instructions). Data from the healthy, younger adults have been presented elsewhere and serves as a basis for this study [9] . Acquisition parameters and experimental design were held constant between older and younger data sets. One younger (31-year-old male) and one older participant (65-year-old male) were excluded from all analyses owing to excessive motion artifacts (>3 mm) within the scanner. In addition, data from one older participant (70-year-old male) was removed from analysis owing to an inability to complete all behavioural blocks because of physical discomfort in the scanner (final total 22 younger and 18 older participants). Neuropsychological testing Before the experiment, older adults were administered a battery of 13 neuropsychological tests (see Supplementary Table 1 ). Participants were required to score within two s.d. of age-matched control values on these tests to be included in the study. The neuropsychological evaluation consisted of tests designed to assess general cognitive function (mini-mental state exam) [67] , verbal learning (CVLT-II), geriatric depression(GDS) [68] , visual-spatial function (modified Rey-Osterrieth figure copy), visual-episodic memory (delayed memory for details of a modified Rey-Osterrieth complex figure, visual-motor sequencing and set-shifting (trail making tests A and B), phonemic fluency (words beginning with the letter ‘D’), semantic fluency (animals), calculation ability (arithmetic), executive functioning, WM and incidental recall backward digit span and digit symbol (WAIS-R). Experimental design The experimental paradigm was comprised of five similar tasks in a delayed-recognition WM task design ( Fig. 1 ), similar to previously published work [9] , [19] . Each task consisted of the same basic temporal sequence with only the instructions differing across tasks. All tasks involved viewing two images (Stim1 and Stim2), each displayed for 800 ms (with a 400-ms inter-stimulus interval (ISI)) followed by a 8-s period (delay) in which the images were to be remembered and mentally rehearsed. After the delay, a third image appeared (probe) for 1,000 s. Each participant was instructed to respond with a button press (as quickly as possible without sacrificing accuracy) whether or not the probe image matched either of the previous two images (Stim1 or Stim2). This was followed by an inter-trial interval lasting 9 s. For three of the five tasks, the Stim1 and Stim2 images were comprised of both a scene and a face superimposed upon each other. Participants were instructed to focus their attention on and remember either the face or the scene, while ignoring the other. In the face memory-overlap task (FM-O), the faces were remembered while the scenes were ignored, and vice versa in the scene memory-overlap task (SM-O). When the probe image appeared, it was composed of an isolated face in the FM-O task, and an isolated scene in the SM-O task. For the passive view (PV-O) task, participants were instructed to view the overlapped images without trying to remember them, after which they responded to an arrow direction (in place of the probe image) with a button press. In this way, the PV-O condition maintains the same visual characteristics as FM-O and SM-O, with only the cognitive goals being changed. For the other two tasks, the Stim1 and Stim2 images were composed of a single stimulus without any distracting/overlapping information: a face in the face-memory task (FM) and a scene in the scene-memory task (SM). The task was presented in blocks of 15 trials with the same condition presented for the entire block. Each condition was presented in two blocks (for a total of 30 trials per condition and 60 total Encode period images per condition), counterbalanced in random order across all participants. Thus, 10 blocks were presented to each participant (2 blocks for each of the 5 conditions), and each block lasted 5 min. Stimuli All stimuli consisted of 225 × 300 pixel grayscale images, presented foveally, subtending a visual angle of 3° from a small cross at the center of the image. The face stimuli consisted of a variety of neutral-expression male and female faces across a large age range. Hair and ears were removed digitally, and a blur was applied along the contours of the face as to remove any potential non-face-specific cues. The gender of the face stimuli was held constant within each trial. Images of scenes were not digitally modified beyond resizing and grayscaling. For the tasks consisting of overlapped faces and scenes, one face and one scene were randomly paired, made transparent and digitally overlapped using Adobe Photoshop CS2 such that both were equally visible. Overlapped and isolated images were randomly assigned to the different tasks. Localizer and default network To identify the visual association cortical region maximally selective to scenes (that is, the PPA) a localizer task independent of the main experimental task was performed, which consisted of 14 interleaved, 12 s blocks of 20 scenes or faces with a 8-s delay between each block [10] . To ensure participant’s maintained vigilance, they were asked to press a button whenever they saw the exact same stimulus presented twice in a row (10% of stimuli presented). fMRI data were acquired and processed as described below. A contrast was created from the GLM β-maps for scenes and faces, and the most active 35 voxels (~0.390 cm 3 ) were selected from the approximate anatomical location for the left PPA (lPPA) [6] , [10] , [21] , [30] . The results from this paper focused solely on the lPPA rather than either FFA or the right PPA. The FFA does not consistently exhibit significant suppression, even in younger adults [10] , [20] , thus previous experiments have utilized only the lPPA for ageing studies [6] . Default network activity was functionally defined as regions where there was greater degree of activity during rest block compared with 1-back task [15] . Group-level contrasts for the default network were performed only on those voxels that showed task-induced deactivations. ROIs for the default network were defined using clusters of activity anatomically constrained to published coordinates of default network nodes [15] , [25] . It should be noted, that the default network was generated via univariate analysis, which technically does not reveal a ‘network’. However, the same set of default regions have also been shown via functional connectivity analysis during a period of a rest [16] . fMRI collection and processing All fMRI data were collected on a Siemens 3T MAGNETOM Treo 3T scanner with stimuli presented on an liquid-crystal display monitor viewed in the prone position by participants using a mirror rigidly attached to the 12-channel head coil. Echoplanar-imaging (EPI) data were acquired (FA=90, TE=25 ms and TR=2 s) with 33 interleaved axial slices (with a 0.5-mm gap) for a final resolution of 1.79 × 1.79 × 3.5 mm per voxel (FOV=23 cm; 128 × 128 matrix). All data preprocessing was conducted in SPM5 (Wellcome Department of Imaging Neuroscience, London, England). Raw blood oxygen level-dependent data were corrected offline for slice-timing acquisition and motion artifacts. To further ensure age-based differences did not arise from group differences in motion artifacts, movement parameters (X, Y, Z, roll, pitch, and yaw) were compared between groups for both mean offset and rate of drift (that is, slope of movement parameters over time). No differences were observed between groups for any of the 12 comparisons (each comparison, P >0.6, corrected). A 5-mm isotropic Gaussian-smoothing kernel was applied using SPM5 before modelling the data. In addition to the EPI data, high-resolution T1-MPRAGE images (1 × 1 × 1 mm voxel size; FOV=160 × 240 × 256 mm, TR=2,300 ms, TE=3 ms and FA=90) were acquired to aid in anatomical localizations of activity and to screen for any undiagnosed neurological trauma. ROI activities were calculated by modelling the encoding (including both stimuli and the inter-stimulus interval), delay periods and probe periods in each condition using a boxcar function convolved with the canonical haemodynamic response function (HRF) for the duration of each epoch as a GLM within SPM5. It should be noted that using a canonical HRF for voxels in all brain regions (including those where the HRF may be a poor descriptor of the underlying data) in a multi-event, multi-trial design may result in brain activity being misattributed to activity in adjacent events [69] . However, all participants from both age groups were modelled with the same approach, and so we do not feel this has impacted our conclusions. Native-space masks for each posterior ROI were created for each participant as described above and the estimated coefficients for encode-period activity were used as a measure of posterior visual associative cortical activations. Analyses focused on left PPA activity owing to its robust measures of suppression, more so than right PPA [6] , [9] , [10] . Group-level univariate analysis was performed by normalizing each participant’s mean EPI image to the MNI (2 × 2 × 2 mm voxel size) template image before Gaussian smoothing and modelling. Voxel-based morphometry analysis Grey-matter volume was modelled by normalizing participants’ T1-MPRAGE images into MNI-normalized space; segmented into grey-matter, white-matter and cerebral spinal fluid maps, and smoothed using a 12-mm isotropic Gaussian kernel in SPM5 as previously described [37] , [38] . All images were manually inspected after segmentation. Correlations were performed on modulated grey-matter images with sex, age and total-intracranial volume as nuisance variables. Resulting images were thresholded at P <0.05 and corrected for multiple comparisons using the method described below. DTI analysis Diffusion tensors (64) were acquired (in addition to one B0 image) at 2.2 × 2.2 × 2.2 mm voxel size, FOV: 220 × 220 mm, Tr=8 s and Te=109 ms. Images were processed using FSL (Analysis Group, FMRIB, Oxford, UK) specifically the FDT and TBSS software packages. TBSS was utilized to project all older participants’ FA data onto a mean group FA tract skeleton. After DTI preprocessing, analysis was performed using voxel-wise cross-subject statistics and adjusted for multiple comparisons using threshold-free cluster enhancement [42] . Network analysis Functional connectivity network maps were created for each participant as described previously using a beta-series correlation analysis approach [22] . The encode, delay and probe stage from each condition and every trial was modelled with its own distinct regressor within the GLM, although only the encode-period activity was analysed. The average value was extracted for each visual associative cortical ROI for each trial and these values were then correlated voxel-wise across the entire brain to find regions with highly revealed regions with co-varying activity across trials with the visual associative cortical ROI. The whole-brain r -value maps for each participant underwent a Fisher’s r to z transformation and the z -values were then normalized to the MNI template and post-normalization Gaussian smoothed (5 mm FWHM) for group level analysis. Group-contrast maps were created by permuting across the condition grouping term (that is, age or suppression) and averaging across the group using 10,000 rounds of permutation [70] . Data were corrected for multiple comparisons by thresholding the P -values at 0.05 and permuting across the expected cluster distribution to find the expected cluster size for P <0.05. Clusters smaller than this value were removed from the analysis. Only positive correlations were considered owing to the overall positive bias in the network analysis method [23] . Whole-brain neural-functional connectivity correlations Correlations between each participant’s index of suppression (encode-period values for the PPA such that FM-O>PV-O conditions) and the degree of functional connectivity between the PPA and every other voxel were performed on MNI-normalized images, thresholded at P <0.05 and corrected for multiple comparisons using the permutation method described in the ‘Network analysis’ section above. Similar analysis was also performed using measures of participants’ distractibility (WM performance on FM–FM-O). Comparative statistics ANOVA’s were utilized throughout analysis using the CLEAVE (‘C Language Exploratory Analysis of Variance with Enhancements’) software package (University of California, Davis) setup as mixed effects analysis (with subject as a random factor, condition as a fixed, within-group factor and age as a fixed, between-group factor) and corrected using the Greenhouse-Geisser method. Post hoc t -tests were corrected for multiple comparisons using Tukey–Kramer’s method and were two-tailed unless specified for checking an a priori analysis. For calculating statistical differences between groups for correlations (that is, Figs 5 and 8 ), a linear regression was calculated for each group along with the s.e. coefficients of the slope. If the two groups did not have overlapping 95% confidence intervals for their slopes, they were judged to be significantly different. How to cite this article: Chadick, J. Z. et al. Structural and functional differences in medial prefrontal cortex underlies distractibility and suppression deficits in ageing. Nat. Commun. 5:4223 doi: 10.1038/ncomms5223 (2014).